Bursting drops in solid dielectrics caused by high voltages Fluid drops tend to be spheres—a shape that minimizes surface energy. In thunderstorm clouds, drops can become unstable and emit thin jets when charged beyond certain limits. The instability of electrified drops in gases and liquids has been widely studied and used in applications including ink-jet printing, electrospinning nanofibers, microfluidics and electrospray ionization. Here we report a different scenario: drops in solids become unstable and burst under sufficiently high electric fields. We find the instability of drops in solids morphologically resembles that in liquids, but the critical electric field for the instability follows a different scaling due to elasticity of solids. Our observations and theoretical models not only advance the fundamental understanding of electrified drops, but also suggest a new failure mechanism of high energy density dielectric polymers, which have diverse applications ranging from capacitors for power grids and electric vehicles to muscle-like transducers for soft robots and energy harvesting. Electrified drops have been intensively studied [1] , [2] , [3] , [4] , [5] , [6] for natural phenomena, such as thunderstorm cloud formation [7] , as well as for technical applications ranging from ink-jet printing [8] , electrospinning nanofibers [9] , [10] , microfluidics [11] to electrospray ionization for assaying biomolecules [12] . It has been known that a strong electric field can destabilize electrified drops in gases and liquids. An unstable drop often deforms into the shape of a cone, referred as Taylor cone, which then emits a stream of smaller drops or a fine jet into the surrounding gas or liquid [1] , [2] , [3] , [4] , [5] , [13] , [14] . The critical electric field for the onset of the Taylor cone scales as , where γ is the surface tension of the drop, R 0 the radius of the drop, and ε the permittivity of the surrounding gas or liquid [1] , [2] , [3] , [4] , [5] , [13] . On the other hand, electrified drops in solids remain largely unexplored, mainly due to the difficulty in observing any relevant phenomenon before electric breakdown of the solids. This limitation not only poses a major challenge in fundamental understanding of electrified drops, but also hampers the development of technology in areas such as high energy density polymer capacitors [15] and muscle-like transducers [16] . Here, we report the first in situ observation of morphological changes of single and multiple drops in solids under electric fields, and present a new theoretical model for the phenomena. We find that the critical electric field for drops in solids to undergo unstable morphological changes follows a scaling different from that for the Taylor cone, and is also significantly affected by the interaction between drops. Our experimental observations and theoretical model further suggest a new failure mechanism for dielectric polymers under electric fields. In situ observation of drops in solids under voltages The experimental setup for observing voltage-induced morphological changes of drops in solids is illustrated in Supplementary Fig. S1 . We fabricated a layer of a soft dielectric polymer (Ecoflex, Smoothon, USA) that traps single or multiple drops of an aqueous solution of sodium chloride or air bubbles. The radius of the drop was set to be much smaller than the thickness of the polymer. The polymer was then sandwiched between two rigid insulating films of fluorinated ethylene propylene (FEP) (McMaster-Carr, USA), coated with transparent electrodes of Pd/Au layers with thickness of 10 nm (see Methods for details on fabrication of the samples). The two electrodes were then subject to a ramping voltage ( Supplementary Fig. S1 ). The rigid films suppress overall deformation and electric breakdown of the dielectric polymer, enabling in situ observation of the drops undergoing morphological changes [17] , [18] . The electric field far away from the drop is uniform and is regarded as the applied electric field, E , on the drop. Two optical microscopes were used to observe the morphological changes of the drops in directions along and normal to the applied electric field ( Supplementary Fig. S1 ). Single drop in solids We first study a single drop of a conductive liquid in polymers. As the electric field ramps up, the drop undergoes a sequence of morphological changes ( Fig. 1a , Supplementary Fig. S2 , Supplementary Movies 1 , and 2 ). The spherical drop deforms into a spheroid gradually, and then becomes unstable suddenly, forming sharp tips on its apexes. The critical electric fields for the formation of sharp tips on two apexes of a drop may be slightly different, due to random factors such as variation of properties of the polymer. This difference makes the drop look asymmetric after the instability ( Fig. 1a ). If the electric field is turned off before or right after the formation of the first sharp tip, the drop will reversibly recover its original shape ( Supplementary Fig. S3 and Supplementary Movie 3 ). On the other hand, if the electric field is further ramped up, the large deformation of the polymer around sharp tips can induce fracture of the polymer. Subsequently, the sharp tips open up, giving the drop a spindle shape. If the electric field further increases, the spindle-shaped drop gradually grows longer and the radius of its centre circle decreases. Eventually, the drop evolves into the shape of a long tube in the polymer ( Supplementary Movie 1 ). If the electric field is turned off at this state, the drop does not recover the original spherical shape; instead, a trace of liquid is trapped along the path of the elongated drop, and the sharp tips at the apexes of the drop remain unrecovered ( Fig. 1b ). The volume of the drop is conserved during the whole process. To our knowledge, this is the first observation of bursting drops in solids under electric fields ( Fig. 1a ; Supplementary Fig. S2 , Supplementary Movies 1 , 2 and 3 ). If the water drop is present in a dielectric polymer under high electric fields, the large deformation and fracture of the polymer can induce failure of the polymer. 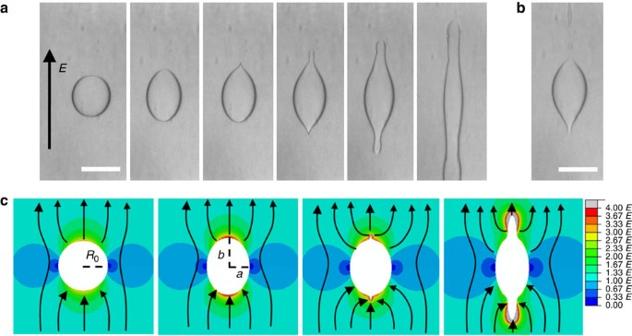Figure 1: Morphological instability of a drop of conductive liquid in a dielectric polymer under electric fields. (a) As the electric field ramps up, the spherical drop gradually deforms into a spheroid, then suddenly forms sharp tips, and eventually evolves into the shape of a tube. The electric fields for panels from left to right are 0, 7.4, 7.7, 9.3, 11, and 18.2 MV m−1. The time for panels from right to left is 0, 98, 102, 123, 145, and 240 s. The scale bar is 100 μm and for all panels. (b) The drop does not recover its original shape after the electric field is turned off. The scale bar is 100 μm. (c) The contours of electric field magnitude around the drops calculated by a finite-element model and the electric-field directions. The local electric field in the polymer is normal to the surface of the drop. The scale bar has a unit of the magnitude of the applied electric field. Figure 1: Morphological instability of a drop of conductive liquid in a dielectric polymer under electric fields. ( a ) As the electric field ramps up, the spherical drop gradually deforms into a spheroid, then suddenly forms sharp tips, and eventually evolves into the shape of a tube. The electric fields for panels from left to right are 0, 7.4, 7.7, 9.3, 11, and 18.2 MV m −1 . The time for panels from right to left is 0, 98, 102, 123, 145, and 240 s. The scale bar is 100 μm and for all panels. ( b ) The drop does not recover its original shape after the electric field is turned off. The scale bar is 100 μm. ( c ) The contours of electric field magnitude around the drops calculated by a finite-element model and the electric-field directions. The local electric field in the polymer is normal to the surface of the drop. The scale bar has a unit of the magnitude of the applied electric field. Full size image The electric-field-induced Maxwell stress drives the morphological changes of the drop in the polymer ( Fig. 1c ) [19] , [20] , [21] , [22] . The Maxwell stress in the polymer can be expressed as where ε is the permittivity of the polymer, E the electric field in the polymer, and I the unit tensor. At the interface between the polymer and the conductive drop, the electric field in the polymer is normal to the interface and is zero inside the conductive drop. Therefore, the Maxwell stress in the polymer gives tractions normal and tangential to the surface of the drop respectively as where n and t are unit vectors normal and tangential to the surface of the drop respectively. Along the applied electric field, the top and bottom apexes of the drop have the highest local electric field ( Fig. 1c ). Therefore, the tractions normal to the surface of the drop tends to elongate the drop along the applied electric field. As the electric field at the apexes reaches a critical value, it causes the formation of the sharp tips [17] . Further increase of the applied electric field causes the drop to elongate into the shape of a tube. The instability of the drops in solids morphologically resembles that of drops in fluids [1] , [2] , [3] , [4] , [5] , [23] , [24] . The scaling for the critical electric field of the Taylor cone in liquids, however, is inapplicable to our observations of the drops in solids. Our experimental observations show that the critical electric fields for the onset of the sharp tips on drops in solids are independent of their radii ( Fig. 2a ). For drops in solids, the Maxwell stress drives the deformation of the drops, which is resisted by both surface tension of the drops and elasticity of the solids. The Maxwell stress in the polymer scales with εE 2 ; the Laplace pressure due to surface tension scales with γ / R 0 ; and the elastic stress in the polymer scales with the shear modulus of the polymer μ . Using typical values of γ ≈4 × 10 −2 Nm −1 , μ ≈4 kPa, and R 0 ≈50~100 μm, we can see that the elastic stress in the polymer is principally responsible for resisting the deformation of the drop. This conclusion suggests a different scaling from that for the Taylor cone. 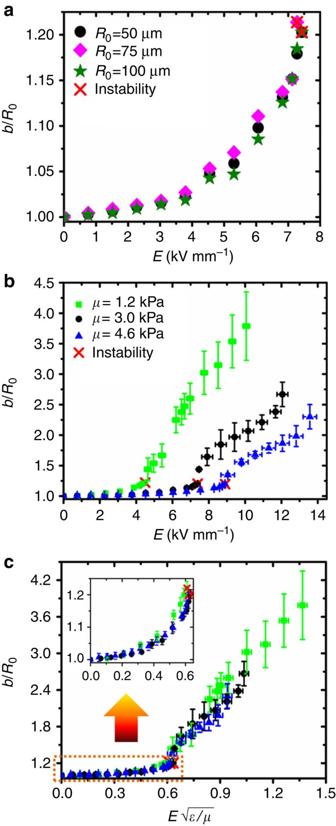Figure 2: Deformation and instability of a single drop of conductive liquid in a dielectric polymer under electric fields. The length of the drop is recorded as a function of the applied electric field. The onset of the first sharp tip is marked by a cross. (a) The curves coincide for drops with different radii ranging from ~50 to ~100 μm in the same polymer. (b) The curves separate for drops in polymers with different moduli (1.2 to 4.6 kPa). (c) The curves for drops in polymers of different moduli coincide again when the electric field is normalized with. The same markers inbandcindicate polymers with the sameμ. Values inbandcrepresent mean and s.d. ofb/R0(n=3–4). A comparison of the Maxwell stress and elastic stress gives that the critical electric field scales as Figure 2: Deformation and instability of a single drop of conductive liquid in a dielectric polymer under electric fields. The length of the drop is recorded as a function of the applied electric field. The onset of the first sharp tip is marked by a cross. ( a ) The curves coincide for drops with different radii ranging from ~50 to ~100 μm in the same polymer. ( b ) The curves separate for drops in polymers with different moduli (1.2 to 4.6 kPa). ( c ) The curves for drops in polymers of different moduli coincide again when the electric field is normalized with . The same markers in b and c indicate polymers with the same μ . Values in b and c represent mean and s.d. of b / R 0 ( n =3–4). Full size image Equation (4) indicates that a stiffer polymer will give a higher critical electric field for the instability of drops in it. It is noted that the strains in polymers do not appear in equation (4), as the deformation of polymers with different moduli and permittivity is the same at the initiation of the instability. To validate equation (4), we prepare samples of the polymer with different shear moduli by changing the crosslink density, and record the length of a drop in each sample as a function of the applied electric field ( Fig. 2b ). The shear modulus of the polymer markedly affects the critical electric field for the formation of sharp tips. When the applied electric field is normalized by , the curves for drops in polymers of different shear moduli coincide ( Fig. 2c ). These experimental results are consistent with the predicted scaling, equation (4). Furthermore, as the evolution of the drop is determined by ( Fig. 2c ), the time scale for the evolution can be evaluated to be , where is the ramping rate of the electric field. Next, we calculate the critical electric field for the onset of the sharp tips. When the applied electric field is small, a drop approximately takes the shape of a spheroid. The local electric field at an apex of a conductive spheroid is [2] , [19] , [25] where b and a are the long and short axes of the spheroid drop, respectively. Right before the formation of the tip, b / a ≈1.33 according to our experimental observation ( Fig. 2c ), and equation (5) gives that E apex ≈3.83 E . To calculate the critical electric field for formation of the sharp tip, we construct an asymmetric finite-element model of the polymer at the apex of the drop ( Supplementary Fig. S4 ) [17] , [18] , [26] , [27] , [28] . Because the size of the tip at initiation is much smaller than the radius of curvature at the apex, we regard the apex as a flat surface under an electric field of E apex . The surface is also under a biaxial stretch of 1.13 to account for the deformation of the drop. At the onset of the sharp tip, the deformation in the polymer is relatively small, and therefore the polymer is taken to follow the ideal neo-Hookean dielectric ( Supplementary Fig. S5 ) [29] . Using the finite-element model, we compare the potential energies of the polymer at the flat and sharp-tip states as a function of E apex . When the potential energy difference between the two states reaches zero, the sharp tip forms (see Supplementary Fig. S6 and Supplementary Methods ). We find that the critical E apex for a sharp tip to form is ( Supplementary Fig. S6 ). Considering E apex ≈3.83 E , the critical applied electric field for onset of the sharp tip can be calculated to be 0.55 . Figure 2c shows that the experimentally measured critical electric field is around 0.33 . The theoretical result matches well with the experimentally measured value. It should be noted that the present theoretical calculation, in contrast to simulations reported in references [23] , [24] on drops in fluids, provides a consistency argument rather than an a priori prediction, because we have used the experimentally observed deformation as boundary conditions in the numerical model. Multiple drops in solids We next study multiple drops in polymers. For simplicity, we will focus on the interaction of two drops in the polymer. The radii of the drops, R a and R b , and the distance between the centres of the drops, d , are set to be on the same order. In several runs of the experiment, we vary the angle between the centre-to-centre vector and the applied electric field, θ . In all cases, when the applied electric field reaches critical values, sharp tips form on one drop in a direction towards the other drop ( Fig. 3 ). The sharp tip usually appears on one drop, instead of simultaneously on both drops. The drop on which the first sharp tip forms can have a larger ( Fig. 3a ) or smaller radius ( Fig. 3b ) than the other one. The interaction of multiple drops in solids morphologically resembles the coalescence of drops in liquids under electric fields [30] , [31] , [32] , [33] , [34] . However, for Taylor cones to form on two drops of equal radius in liquids, the initial distance between the centres of the drops needs to be greater than ~3.2 times of the radius [33] . On the other hand, we have not observed such a critical distance for onset of sharp tips on drops in solids (for example, Fig. 3 ). 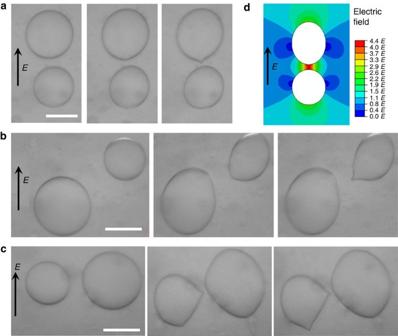Figure 3: Deformation and instability of two drops in a polymer under electric fields. The angle between the centre-to-centre vector of drops and the applied electric field,θ, is set to be (a) 0°, (b) 45° and (c) 90°. (d) The contours of electric field magnitude around the two drops in (a) calculated by a finite-element model. The scale bar is 100 μm ina,bandc. The scale bar indhas a unit of the magnitude of the applied electric field. Figure 3: Deformation and instability of two drops in a polymer under electric fields. The angle between the centre-to-centre vector of drops and the applied electric field, θ , is set to be ( a ) 0°, ( b ) 45° and ( c ) 90°. ( d ) The contours of electric field magnitude around the two drops in ( a ) calculated by a finite-element model. The scale bar is 100 μm in a , b and c . The scale bar in d has a unit of the magnitude of the applied electric field. Full size image The formation of tips in two drops in solids is also different from that in a single drop in solids, because the interaction of drops significantly enhances local electric fields in regions between them ( Fig. 3d ). As a result, the first tip tends to form on one drop along a direction towards the other one ( Fig. 3 ). Furthermore, the critical electric field for the onset of the tip in two drops can be significantly lower than that for a single drop in the same polymer. For instance, the critical field is in Fig. 3a , in Fig. 3b and in Fig. 3c . Considering equation (4), we express the critical field for the onset of sharp tips in two drops as: where Z is a non-dimensional parameter that accounts for the geometry and interaction of the two drops. If d / R a approaches infinity, we recover the single-drop case with Z =0.55. Following a similar procedure ( Supplementary Fig. S7 ), we calculate the critical field for the two drops in Fig. 3a to be , which matches well with the experimental result. In Supplementary Fig. S8 , we plot the enhancement of the electric field in a polymer with two spherical drops of equal size as a function of their distance d / R a and the orientation of the electric field θ [35] . It can be seen that the minimum enhancement of the electric field is three times when d / R a approaches infinity (that is, the single-drop case). When the distance between the drops decreases, the enhancement of the electric field increases. A higher enhancement of the electric field can give a lower critical electric field for the instability. We note that the critical electric fields for the onset of sharp tips on drops in dielectric polymers are significantly lower than those for two other modes of electromechanical instabilities: the pull-in instability (refs 36 , 37 ) and the electro-creasing instability [17] . Furthermore, after forming sharp tips the drops elongate drastically, potentially inducing electric breakdown of the polymer ( Fig. 1 ). Our experimental observations and physical model suggest a new failure mechanism for dielectric polymers under electric fields: defects such as cavities and water drops can initiate sharp tips in polymers under electric fields and subsequently cause breakdown of the polymers. To test the hypothesis, we measure the breakdown field of a silicone rubber (Ecoflex, Smoothon, USA) with various volume ratios of water drops. Polymer films with three different moduli are mounted between a copper plate and a copper rod, which can suppress the pull-in and electro-creasing instabilities ( Supplementary Fig. S9 ) [27] . A direct current voltage is applied between the rod and the plate until electrical breakdown of the film. The measured breakdown fields for films with various moduli are given in Fig. 4a . The breakdown field can be significantly reduced by a very low volume concentration of drops (for example, 1%), where the distances between drops are much larger than their sizes (that is, the single-drop case). The breakdown field further decreases with the increase of drop concentration, as the drops begin to interact with one another ( Fig. 4a ). Furthermore, the breakdown field approximately scales with , indicating the instability of drops induces breakdown of the polymer. 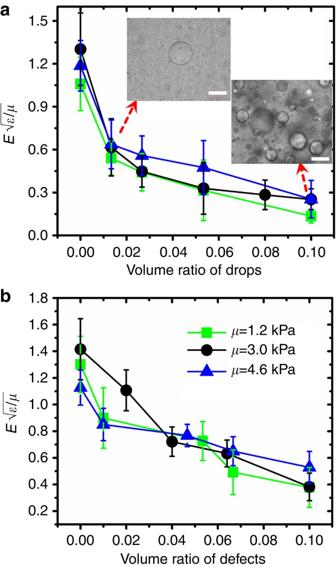Figure 4: The effect of water drops and air bubbles on the breakdown electric field of a polymer. Both (a) water drops and (b) air bubbles can significantly reduce the breakdown electric field of the polymer. The scale bar is 100 μm ina. Values inaandbrepresent mean and s.d. of breakdown fields (n=10–20). Figure 4: The effect of water drops and air bubbles on the breakdown electric field of a polymer. Both ( a ) water drops and ( b ) air bubbles can significantly reduce the breakdown electric field of the polymer. The scale bar is 100 μm in a . Values in a and b represent mean and s.d. of breakdown fields ( n =10–20). Full size image In addition, we replace water drops in the polymers with air bubbles and repeat the above breakdown tests. The breakdown field also decreases with the increase of volume concentration of bubbles and approximately scales with ( Fig. 4b ). As air is not conductive, the electric field in air bubbles is not zero. The electric-field-induced Maxwell stress in an air bubble can be expressed as where ε 0 is the permittivity of air. The Maxwell stress in the polymer and the air bubble gives tractions normal and tangential to the surface of the bubble respectively as where E n and E t are the electric fields, in the polymer, normal and tangential to the bubble surface respectively. Due to symmetry, E t =0 at the apexes of the bubble and thus . As the permittivity of the polymer is higher than that of air (that is, ε > ε 0 ), the traction tends to deform the air bubble into an oblate spheroid that may undergo instabilities. It should be noted that we have assumed the polymer is a perfect dielectric with zero conductivity. For drops with lower permittivity in liquids with higher permittivity under electric fields, the shapes of the drops can become either prolate or oblate depending on the permittivity and conductivity of the liquids [14] , [38] . In addition, in the current study, the elastic stress in the polymer is principally responsible for resisting the deformation of the air bubbles, leading to the scaling in Fig. 4b . From the above analyses, it is evident that dielectric polymers with higher moduli and fewer defects will have higher breakdown fields if the instability induces electrical breakdown of the polymers. In many cases, however, it is desirable to make dielectric polymers with low moduli for functions such as large actuation strains [39] . To increase breakdown fields while maintaining low moduli of polymers, one may enhance the fracture toughness and stiffening properties of the polymers to prevent the evolution of the instability [29] (that is, from sharp tip to tube in Fig. 1a ). If the drops cease to elongate after the formation of sharp tips, the breakdown field of the polymer may be enhanced. In summary, we present the first in situ observation of morphological instability of single and multiple drops in solids under electric fields. A single drop in solids first forms a sharp tip that resembles a Taylor cone in liquids, and then evolves into the shape of a long tube. The critical electric field for the onset of sharp tips in solids follows a scaling different from that for the Taylor cone, owing to the elasticity of the solids. Multiple drops in solids under electric fields also form sharp tips. The critical field for the onset of the sharp tips in multiple drops can be significantly reduced due to the interaction between the drops. Our observations and theoretical models not only advance the fundamental understanding of electrified drops, but also suggest a new failure mechanism of high energy density dielectric polymers, which are under intense development for applications ranging from capacitors for power grids and electric vehicles [15] , [16] to muscle-like transducers for soft robots and energy harvesting [15] , [16] , [40] , [41] , [42] . Sample preparation To fabricate samples that contain conductive drops, a conductive liquid (10% wt sodium chloride solution) was uniformly mixed with uncrosslinked solution of a silicone elastomer Ecoflex 00-10 (Smoothon, USA) with volume concentration ranging from 1 to 10%. After mixing, many water drops with radii from 50 to 100 μm were trapped inside the polymer solution. The polymer solution was then cast into films of thickness of 1.2 mm, and cured at 60 °C for an hour. The volume ratio of crosslinker and base of Ecoflex was varied from 0.1:1 to 0.5:1 to obtain polymers with shear moduli ranging from 1.2 to 4.6 kPa. A rigid transparent polymer film FEP (McMaster-Carr, USA) with a thickness of 50 μm and modulus over 1 GPa were attached to both sides of the Ecoflex films. Pd/Au layers with a thickness of 10 nm (Sputter Coater, Denton Vacuum, USA) were coated on the FEP film as electrodes. To fabricate samples with air bubbles, drops of deionized water were embedded in the polymer. The samples were then baked in an oven at 60 °C for 12 h with the water drops evaporated. Observation of drop evolution Supplementary Fig. S1 illustrates the experimental setup for in situ observation of the evolution of drops in polymers under electric fields. A direct current voltage was applied between the two electrodes with a ramping rate of 100 Vs −1 using a high-voltage supply (Matsusada, Japan). One or two drops far away from others and the surfaces of the elastomer were chosen to be observed from microscope objectives (Nikon, Japan) normal to and along the applied electric field. The evolution of the drop under the applied electric field was recorded by cameras on the microscope. When the sharp tip formed at the end of the drop, the voltage was recorded as the critical voltages φ c . The critical electric fields were calculated by , where H is the thickness of Ecoflex film, H s is the thickness of FEP film, ε =2.5 ε 0 and ε s =2.1 ε 0 are the dielectric permittivity of Ecoflex, and ε 0 =8.85 × 10 −12 Fm −1 is the permittivity of vacuum. Breakdown test The breakdown fields of Ecoflex films with 1 mm thickness were measured using the experimental setup demonstrated in Supplementary Fig. S9 . The Ecoflex film was bonded on a copper substrate and immersed in silicone oil (Robinair, USA). A metal rod with a spherical tip of 8 mm in diameter was constrained to prevent movement, and placed vertically in touch with the Ecoflex film. A controllable ramping voltage was applied between the rod and the substrate until electrical breakdown. Numerical calculation To calculate the critical electric field for the onset of the sharp tip, finite-element software, ABAQUS 6.10.1 was used to analyse the deformation and electric field of the polymer at the apex of the drop ( Supplementary Fig. S6 ) [17] . The programme code is validated by benchmark calculations and the mesh accuracy is ascertained through a mesh refinement study. The region is taken to deform under axisymmetric conditions, and obey the neo-Hookean and ideal dielectric laws [29] . How to cite this article: Wang, Q. et al . Bursting drops in solid dielectrics caused by high voltages. Nat. Commun. 3:1157 doi: 10.1038/ncomms2178 (2012).